Stk38 protein kinase preferentially inhibits TLR9-activated inflammatory responses by promoting MEKK2 ubiquitination in macrophages NDR/LATS kinase family is highly conserved from yeast to human. It remains unknown whether the members of this family function in innate immune responses. Here we demonstrate that Stk38 negatively regulates TLR9-mediated immune responses in macrophages. Stk38 constitutively associates with ubiquitin E3 ligase Smurf1, and facilitates Smurf1-mediated MEKK2 ubiquitination and degradation. MEKK2 is required for CpG-induced ERK1/2 activation, TNF-α and IL-6 production but not required for LPS-induced TNF-α and IL-6 production. Accordingly, Stk38 deficiency increases CpG-induced ERK1/2 activation, TNF-α and IL-6 production without significantly affecting LPS-induced TNF-α and IL-6 production. Stk38-deficient mice produce more TNF-α and IL-6, and display increased lethality than control wild-type mice upon E. coli infection. Stk38-deficient mice are also more susceptible to CLP-induced sepsis than control mice. Thus, Stk38 is important in limiting inflammatory cytokine production and necessary for protecting host from inflammatory injury during infection, possibly by negatively regulating TLR9 signalling. Toll-like receptors (TLRs), expressed mainly in innate immune cells, function as key sentinel receptors for invading pathogens to initiate innate immunity and regulate subsequent adaptive immunity [1] . Members of TLR family recognize different conserved pathogen-associated molecule patterns. For example, TLR2 recognizes lipoteichoic acid (LTA), TLR4 recognizes lipopolysaccharide (LPS), TLR9 recognizes CpG oligodeoxynucleotide motif in bacteria and TLR3 recognizes double-stranded RNA from virus. Among TLR family members, TLR2, TLR5, TLR7, TLR8 and TLR9 activate MyD88 (myeloid differentiation primary response gene 88)-dependent signal transduction. TLR3 activates TRIF (Toll/IL-1 receptor domain containing adaptor inducing IFN-β)-dependent signal transduction, and TLR4 activates both MyD88- and TRIF-dependent signal pathways. Both of the MyD88 and TRIF pathways activate nuclear factor (NF)-κB and mitogen-activated protein kinases (MAPKs) to induce inflammatory cytokine production [2] . However, upon recognizing diverse pathogen-associated molecule patterns, TLR family members trigger production of different cytokine profiles and induce different immune responses. Although TLR2 activation facilitates Th2 adaptive immune responses, TLR9 activation facilitates Th1 adaptive immune responses. These observations indicate that TLR family members trigger different downstream signal transduction events. It remains not clear how the signals of TLR family members are differently activated and regulated. Members of MAP3K family, including tumour growth factor-activated kinase 1 (TAK1, MAP3K7), tumour progression locus 2 (Tpl2, MAP3K8), apoptosis signal-regulating kinase 1 (ASK1, MAP3K5), MEKK1 (MAP3K1) and MEKK3 (MAP3K3), have been proven to play important but different roles in TLR signal transduction downstream of MyD88 and TRIF adaptor proteins. Tak1 (MAP3K7) is essential for NF-κB activation in the signal transduction of all of the known TLR family members [3] . Tpl2 activates ERK1/2 in TLR4 signllaing [4] . ASK1 is crucial for activation of p38 pathway in the signalling of TLR4, but not other TLRs [5] . MEKK1 is critical for JNK activation but inhibits ERK1/2 activation in LPS- and double-stranded RNA-induced TLR signalling [6] . MEKK3 deficiency significantly suppresses TLR4-mediated JNK, p38 and NF-κB activation and subsequent inflammatory cytokine interleukin (IL)-6 production in MEF, but it only slightly affects TLR9-mediated JNK activation [7] . MEKK2 is a MAP3K family member closely related to MEKK3 in MEKK/STE11 subfamily. It was reported that MEKK2 was associated with TRAF6 and phosphorylated following LPS stimulation in RAW264.7 cells, and overexpression of MEKK2(S519A) mutant inhibited LPS-induced Elk1 luciferase reporter gene expression in the cells, suggesting that MEKK2 might be involved in TLR4 signal transduction [8] . However, overexpression of MEKK2 did not affect LPS-induced cathelicidin-related antimicrobial peptide gene expression in mast cells [9] . The exact role of endogenous MEKK2 in TLR-mediated immune responses requires further investigation. Moderate activation of TLRs is necessary for host defence against invading pathogens. But excessive activation of TLR signalling and production of proinflammatory cytokines might result in immunological diseases and even development of cancer [10] , [11] . To avoid these unexpected conditions, immune cells develop multiple mechanisms to restrict TLR signal transduction. Many molecules have been found to negatively regulate TLR signalling, ranging from extracellular decoy receptors to intracellular inhibitors [12] . In a recent study, histone methyltransferase Ash1l was found to suppress TLR-triggered inflammatory cytokine production and Ash1l-silenced mice were more susceptible to autoimmune disease [13] . Although intensively studied, the mechanisms by which TLR signal transduction is activated and regulated have not yet been fully understood. Serine/threonine kinase 38 (Stk38), also known as nuclear Dbf2p-related kinase 1 (Ndr1), is a member of NDR/LATS kinase family, a subfamily of the AGC group of serine/threonine kinases, highly conserved from yeast to man. Stk38 is required for proper centrosome duplication [14] . Stk38 promotes Fas-induced apoptosis [15] . Ablation of Stk38 predisposes mice to develop T-cell lymphoma [16] . Stk38 also promotes cell cycle G1 progression by stabilizing c-myc and preventing p21 accumulation [17] . By now, the role of Stk38 in immune responses remains unknown. In the present study, we identify MEKK2 as a positive regulator of TLR9 signalling and Stk38 as a negative regulator of TLR9 signalling in macrophages. MEKK2 knockdown impairs CpG-induced ERK1/2 activation and significantly inhibits CpG-induced proinflammatory cytokine production but not LPS- and LTA-induced proinflammatory cytokine production in macrophages. Stk38 constitutively associates with SMAD (small mothers against decapentaplegic)-specific E3 ubiquitin protein ligase 1 (Smurf1), promotes Smurf1-mediated K48-linked ubiqitination of MEKK2 and inhibits MEKK2 expression. Consistent with the role of MEKK2 in TLR signalling, Stk38 deficiency increases CpG-induced ERK1/2 activation and proinflammatory cytokine production without significantly affecting LPS- and LTA-induced proinflammatory cytokine production in macrophages. Stk38 deficiency also increases CpG-induced proinflammatory cytokine production in vivo . Stk38-deficient mice produce more proinflammatory cytokines and display increased mortality upon bacterial infection than control mice. Stk38-deficient mice are also more susceptible to cecal ligation and puncture (CLP)-induced polymicrobial sepsis than control mice, demonstrating that Stk38 is important for protecting host from TLR9 activation-mediated inflammatory injury. Stk38 inhibits TLR9-mediated inflammatory responses To identify new regulators of TLR signalling, we utilized small interfering RNAs (siRNAs) to screen molecules that could affect LPS- or CpG-induced IL-6 mRNA expression in mouse peritoneal macrophages. We found that siRNA targeting Stk38 significantly increased CpG-induced IL-6 production ( Supplementary Fig. 1 ). To further investigate the role of Stk38 in TLR-mediated inflammatory responses, we transfected RAW264.7 cells with vectors expressing short hairpin RNA (shRNA) specific for Stk38 and control shRNA, and generated cell line in which Stk38 expression was stably inhibited ( Supplementary Fig. 2 ). After TLR agonists challenge, IL-6 production in the supernatant of the cells was detected. As shown in Fig. 1a , Stk38 knockdown marginally affected LPS- and LTA-induced IL-6 production but remarkably increased CpG-induced IL-6 production. We compared the effects of Stk38 knockdown on LPS- and CpG-induced IL-6 and tumour necrosis factor (TNF)-α mRNA expression. Stk38 knockdown slightly increased LPS-induced TNF-α and IL-6 mRNA expression but robustly increased CpG-induced TNF-α and IL-6 mRNA expression ( Fig.1b ). 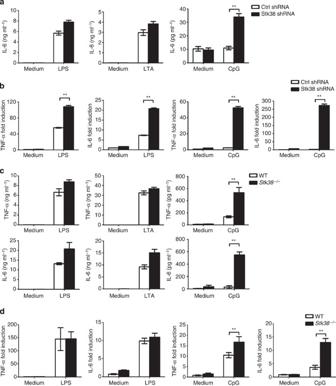Figure 1: Stk38 deficiency increases TLR9-mediated inflammatory responses. (a) ELISA assay of IL-6 in the supernatants of RAW264.7 cells stably transfected with Stk38 shRNA and control (Ctrl) vector, stimulated with 100 ng ml−1LPS, 5 μg ml−1LTA or 10 μg ml−1CpG for 6 h. Data are shown as mean±s.d. (n=3). **P<0.01 (Student’st-test). Similar results were obtained in three independent experiments. (b) Cells as inawere stimulated with 100 ng ml−1LPS or 10 μg ml−1CpG for 1.5 h. TNF-α and IL-6 mRNA expression in the cells was detected by real-time PCR. Data are shown as mean±s.d. (n=3). **P<0.01 (Student’st-test). Similar results were obtained in three independent experiments. (c) ELISA assay of TNF-α and IL-6 in the supernatants of wild-type (WT) and Stk38-deficient (Stk38−/−) mouse peritoneal macrophages stimulated with 100 ng ml−1LPS, 5 μg ml−1LTA or 10 μg ml−1CpG for 6 h. Data are shown as mean±s.d. (n=3). **P<0.01 (Student’st-test). Similar results were obtained in three independent experiments. (d) Wild-type (WT) and Stk38-deficient (Stk38−/−) mouse peritoneal macrophages were stimulated with 100 ng ml−1LPS or 10 μg ml−1CpG for 1.5 h. TNF-α and IL-6 mRNA expressions were detected by real-time PCR. Data are shown as mean±s.d. (n=3). **P<0.01 (Student’st-test). Similar results were obtained in three independent experiments. Figure 1: Stk38 deficiency increases TLR9-mediated inflammatory responses. ( a ) ELISA assay of IL-6 in the supernatants of RAW264.7 cells stably transfected with Stk38 shRNA and control (Ctrl) vector, stimulated with 100 ng ml −1 LPS, 5 μg ml −1 LTA or 10 μg ml −1 CpG for 6 h. Data are shown as mean±s.d. ( n =3). ** P <0.01 (Student’s t -test). Similar results were obtained in three independent experiments. ( b ) Cells as in a were stimulated with 100 ng ml −1 LPS or 10 μg ml −1 CpG for 1.5 h. TNF-α and IL-6 mRNA expression in the cells was detected by real-time PCR. Data are shown as mean±s.d. ( n =3). ** P <0.01 (Student’s t -test). Similar results were obtained in three independent experiments. ( c ) ELISA assay of TNF-α and IL-6 in the supernatants of wild-type (WT) and Stk38-deficient ( Stk38 −/− ) mouse peritoneal macrophages stimulated with 100 ng ml −1 LPS, 5 μg ml −1 LTA or 10 μg ml −1 CpG for 6 h. Data are shown as mean±s.d. ( n =3). ** P <0.01 (Student’s t -test). Similar results were obtained in three independent experiments. ( d ) Wild-type (WT) and Stk38-deficient ( Stk38 −/− ) mouse peritoneal macrophages were stimulated with 100 ng ml −1 LPS or 10 μg ml −1 CpG for 1.5 h. TNF-α and IL-6 mRNA expressions were detected by real-time PCR. Data are shown as mean±s.d. ( n =3). ** P <0.01 (Student’s t -test). Similar results were obtained in three independent experiments. Full size image To rule out the regulatory role of Stk38 knockdown described above was due to off-target effects of the used interfering RNAs, we isolated primary peritoneal macrophages from Stk38 gene knockout mice and control wild-type littermates to observe the effects of Stk38 deficiency on LPS-, LTA- and CpG-induced proinflammatory cytokine production. As shown in Fig. 1c , Stk38 deficiency did not significantly affect LPS- or LTA-induced TNF-α and IL-6 production in peritoneal macrophages. However, CpG-induced TNF-α and IL-6 productions were remarkably increased in Stk38-deficient peritoneal macrophages compared with that in wild-type control cells. Stk38 deficiency did not affect LPS-induced TNF-α and IL-6 mRNA expression but significantly increased CpG-induced TNF-α and IL-6 mRNA expression ( Fig. 1d ). These results demonstrated that Stk38 preferentially inhibited TLR9-mediated inflammatory responses in macrophages. NDR kinases are highly homologous and are reported to have similar functions such as regulating G(1)/S cell transition. We examined the function of Stk38L (NDR2) in TLR9-activated signalling. Knockdown of Stk38L with siRNA increased CpG-induced IL-6 expression ( Supplementary Fig. 3 ), suggesting that NDR2/STK38L had similar functions with NDR1 in regulating TLR9-activated signalling. To explore the role of Stk38 in innate immune responses against bacterial infection, Stk38 knockout mice and wild-type control mice were challenged by peritoneal administration of Escherichia coli ( E. coli ). After E. coli infection, 80% of Stk38-deficient mice died within 18 h, meanwhile, all of the wild-type control mice were still alive. Thirty hours after E. coli infection, all of the Stk38-deficient mice died, in contrast, 60% of the wild-type control mice were still alive ( Fig. 2a ). TNF-α and IL-6 concentrations in the serum of Stk38-deficient mice were much higher than that in the serum of wild-type control mice after E. coli infection ( Fig. 2b ), suggesting that the increased mortality of Stk38-deficient mice might be due to higher proinflammatory cytokine production. Polymicrobial sepsis in mouse experimental peritonitis model induced by CLP was previously shown to be TLR9 dependent [18] , [19] . We used this model to validate the function of Stk38 in TLR9-mediated innate immunity in vivo . After CLP surgery, Stk38-deficient mice displayed worse disease score ( Fig. 2c ), earlier and increased mortality ( Fig. 2d ). We also examined the role of TLR4 in CLP-induced sepsis. Following CLP surgery, mortality and serum levels of TNF-α and IL-6 were similar in TLR4 knockout mice and wild-type mice ( Supplementary Fig. 4 ), suggesting that TLR4 activation was irrelevant with CLP-induced sepsis. To confirm the role of Stk38 in TLR9 signalling in vivo , Stk38-deficient mice and control mice were intraperitoneally injected with CpG and then levels of TNF-α and IL-6 in the serum were detected. Stk38-deficient mice produced more IL-6 and TNF-α than wild-type control mice ( Fig. 2e ). Meanwhile, serum TNF-α and IL-6 levels in Stk38-deficient mice after thioglycollate treatment and LPS challenge were comparable to that in wild-type mice ( Supplementary Fig. 5 ). These results demonstrated that Stk38 functioned as a negative regulator of TLR9 signalling in vivo . 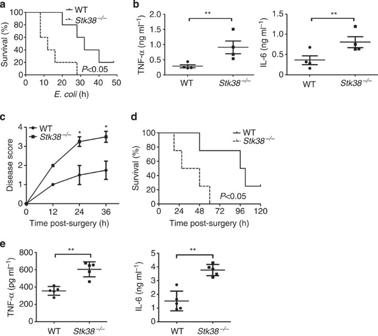Figure 2: Stk38 protects host from TLR9-triggered inflammation. (a) The survival rates of wild-type (WT) and Stk38-deficient (Stk38−/−) mice were monitored for 2 days after intraperitoneally infected with 5 × 107liveE. coli(strain O111:B4; seven to eight mice per phenotype,P<0.05, Gehan–Breslow–Wilcoxon test). Data are representative of three independent experiments with similar results. (b) ELISA assay of TNF-α and IL-6 in serum of wild-type (WT) and Stk38-deficient (Stk38−/−) mice intraperitoneally infected with 5 × 107liveE. coli(strain O111:B4) for 6 h (n=4 per phenotype). **P<0.01 (Student’st-test). Data are representative of three independent experiments with similar results. (c) Clinical symptoms in CLP surgery mice were scored as follows: 0=bright, alert, responsive; 1=slightly lethargic; 2=lethargic and hunched; 3=very lethargic, hunched and shaky; 4=dead (four mice per phenotype). Four mice per phenotype,*P<0.05 (Student’st-test). Data are representative of two independent experiments with similar results. (d) Survival rates of WT and Stk38-deficient (Stk38−/−) mice were monitored for 5 days after CLP (four mice per phenotype,P< 0.05, Gehan–Breslow–Wilcoxon test). Data are representative of two independent experiments with similar results. (e) ELISA assay of TNF-α and IL-6 in serum of WT and Stk38-deficient (Stk38−/−) mice, intraperitoneally injected with thioglycollate to elicite macrophages and then stimulated by intraperitoneal injection of 50 μg CpG for 2 h. Error bars represent s.d. Five mice per phenotype,**P<0.01 (Student’st-test). Data were from two independent experiments. Figure 2: Stk38 protects host from TLR9-triggered inflammation. ( a ) The survival rates of wild-type (WT) and Stk38-deficient ( Stk38 −/− ) mice were monitored for 2 days after intraperitoneally infected with 5 × 10 7 live E. coli (strain O111:B4; seven to eight mice per phenotype, P <0.05, Gehan–Breslow–Wilcoxon test). Data are representative of three independent experiments with similar results. ( b ) ELISA assay of TNF-α and IL-6 in serum of wild-type (WT) and Stk38-deficient ( Stk38 −/− ) mice intraperitoneally infected with 5 × 10 7 live E. coli (strain O111:B4) for 6 h ( n =4 per phenotype). ** P <0.01 (Student’s t -test). Data are representative of three independent experiments with similar results. ( c ) Clinical symptoms in CLP surgery mice were scored as follows: 0=bright, alert, responsive; 1=slightly lethargic; 2=lethargic and hunched; 3=very lethargic, hunched and shaky; 4=dead (four mice per phenotype). Four mice per phenotype,* P <0.05 (Student’s t -test). Data are representative of two independent experiments with similar results. ( d ) Survival rates of WT and Stk38-deficient ( Stk38 −/− ) mice were monitored for 5 days after CLP (four mice per phenotype, P < 0.05, Gehan–Breslow–Wilcoxon test). Data are representative of two independent experiments with similar results. ( e ) ELISA assay of TNF-α and IL-6 in serum of WT and Stk38-deficient ( Stk38 −/− ) mice, intraperitoneally injected with thioglycollate to elicite macrophages and then stimulated by intraperitoneal injection of 50 μg CpG for 2 h. Error bars represent s.d. Five mice per phenotype,** P <0.01 (Student’s t -test). Data were from two independent experiments. Full size image In a recent study, whole-blood samples were collected daily for up to 5 days from patients admitted to the intensive care unit with sepsis, and RNA isolated from the samples was assayed by microarray analysis [20] , [21] . By consulting the deposited GEO data set, we compared Stk38 gene expressions between survival and non-survival patients in the study. Stk38 expression level in whole blood from non-survivors was constantly lower than that of survivors during the first 3 days after their admission to the intensive care unit ( Supplementary Fig. 6 , data accessible at NCBI GEO database, accession GSE54514 , ID:108617105), suggesting that the expression level of Stk38 might correlate with clinical severity of sepsis and play a guiding role for the clinical immunotherapy. Stk38 inhibits TLR9-mediated ERK1/2 activation TLR agonists induce proinflammatory cytokine production by activating MAPK and NF-κB pathways. To investigate the mechanism by which Stk38 negatively regulated TLR9-induced proinflammatory cytokine production, we observed the effects of Stk38 deficiency on CpG-induced MAPK and NF-κB activation in peritoneal macrophages. As shown in Fig. 3a , Stk38 deficiency greatly enhanced CpG-induced ERK1/2 phosphorylation without affecting CpG-induced p38, JNK and NF-κB p65 phosphorylation. Meanwhile, Stk38 deficiency only slightly increased LPS-induced ERK1/2 activation ( Fig. 3b ). These results demonstrated that Stk38 negatively regulated CpG-induced proinflammatory cytokine production by inhibiting ERK1/2 pathway activation. TLR9 activates ERK1/2 through MyD88-dependent pathway. We observed the effect of Stk38 overexpression on MyD88-induced Elk1 luciferase reporter gene expression. HEK293T cells were transfected with vectors expressing MyD88 together with vector expressing luciferase reporter gene controlled by Elk1 and indicated doses of vector expressing Stk38. As shown in Fig. 3c , MyD88 overexpression activated Elk1 reporter gene expression. Stk38 dose-dependently inhibited MyD88-induced Elk1 luciferase reporter gene expression, providing further evidence that Stk38 could inhibit ERK1/2 activation in TLR signal transduction. 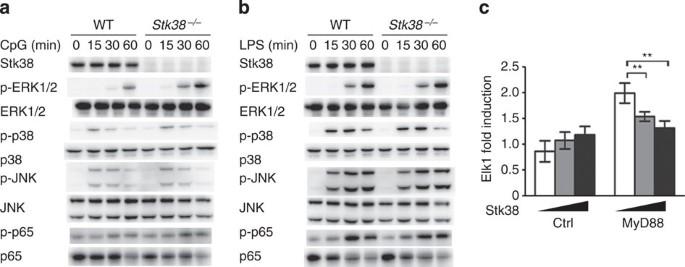Figure 3: Stk38 inhibits TLR9-mediated ERK1/2 activation. (a,b) Peritoneal macrophages from wild-type and Stk38-deficient mice were stimulated with 10 μg ml−1CpG (a) or 100 ng ml−1LPS (b) for indicated time. Phosphorylated and total ERK1/2, p38, JNK and NF-κB p65 were detected by western blot. Similar results were obtained in three independent experiments. (c) HEK 293T cells were transfected with 50 ng MyD88-expressing plasmid, 100 ng Elk1 luciferase reporter plasmid, 2.5 ng pTK-Renilla-luciferase, together with 0, 100 or 200 ng of Stk38-expressing plasmid. Total amounts of plasmid DNA were equalized using control (Ctrl) empty vector. After 24 h of culture, luciferase activity was measured and normalized byRenillaluciferase activity. Data are shown as mean ±s.d. (n=4) of one typical experiment (**P<0.01, Student’st-test). Similar results were obtained in three independent experiments. Figure 3: Stk38 inhibits TLR9-mediated ERK1/2 activation. ( a , b ) Peritoneal macrophages from wild-type and Stk38-deficient mice were stimulated with 10 μg ml −1 CpG ( a ) or 100 ng ml −1 LPS ( b ) for indicated time. Phosphorylated and total ERK1/2, p38, JNK and NF-κB p65 were detected by western blot. Similar results were obtained in three independent experiments. ( c ) HEK 293T cells were transfected with 50 ng MyD88-expressing plasmid, 100 ng Elk1 luciferase reporter plasmid, 2.5 ng pTK-Renilla-luciferase, together with 0, 100 or 200 ng of Stk38-expressing plasmid. Total amounts of plasmid DNA were equalized using control (Ctrl) empty vector. After 24 h of culture, luciferase activity was measured and normalized by Renilla luciferase activity. Data are shown as mean ±s.d. ( n =4) of one typical experiment (** P <0.01, Student’s t -test). Similar results were obtained in three independent experiments. Full size image MEKK2 mediates ERK1/2 activation in TLR9 signalling Stk38 was reported to inhibit MEKK2-induced JNK activation [22] . This promoted us to investigate the role of MEKK2 in TLR-mediated immune responses. We used MEKK2-specific siRNA to inhibit endogenous MEKK2 in mouse peritoneal macrophages ( Fig. 4a ). MEKK2 siRNA slightly inhibited LPS-induced TNF-α and IL-6 production ( Fig. 4b ). In contrast, MEKK2 siRNA significantly inhibited CpG-induced TNF-α and IL-6 production ( Fig. 4b ). Consistently, MEKK2 siRNA remarkably inhibited CpG-induced TNF-α and IL-6 mRNA expression ( Fig. 4c ). To illuminate the role of MEKK2 in TLR-activated inflammatory cytokine production, we used another MEKK2-specfic siRNA (MEKK2 siRNA2) to inhibit MEKK2 expression. MEKK2 siRNA2 also inhibited CpG-induced IL-6 production but did not significantly affect LPS- and LTA-induced IL-6 production, providing additional evidence that MEKK2 is important for TLR9 signalling ( Supplementary Fig. 7 ). The effects of MEKK2 knockdown on LPS- and CpG-induced MAPK and NF-κB activation were detected by western blot. Consistently with the effects of Stk38 deficiency, MEKK2 knockdown remarkably inhibited CpG-induced ERK1/2 activation without affecting CpG-induced p38, JNK and NF-κB activation ( Fig. 4d ). In contrast, MEKK2 knockdown only slightly affected LPS-induced ERK1/2 activation ( Fig. 4e ). We also observed the effects of MEKK2 overexpression on MyD88-induced Elk1 activation. We constructed wild-type MEKK2-expressing plasmid and mutant MEKK2ΔC plasmid, which included MEKK2 N-terminal 1-351 amino acids and lacked C-terminal kinase domain. As shown in Fig. 4f , overexpression of wild-type MEKK2 increased MyD88-induced Elk1 luciferase reporter gene expression. In contrast, MEKK2ΔC inhibited MyD88-induced Elk1 luciferase reporter gene expression. These results demonstrated that MEKK2 was a mediator of TLR9 signalling and was required for TLR9-mediated ERK1/2 activation and proinflammatory cytokine production in macrophages. 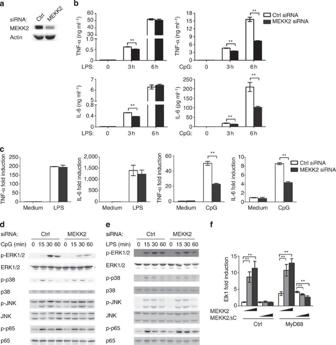Figure 4: MEKK2 mediates ERK1/2 activation in TLR signalling. (a) Immunoblot assay of MEKK2 expression in mouse peritoneal macrophages transfected with 30 nM control siRNA (Ctrl) or MEKK2 siRNA. Similar results were obtained in three independent experiments. (b) ELISA assay of TNF-α and IL-6 in the supernatants of the cells transfected as inaand then stimulated with 100 ng ml−1LPS or 10 μg ml−1CpG for 6 h. Data are shown as mean±s.d. (n=3). **P<0.01 (Student’st-test). Similar results were obtained in three independent experiments. (c) Real-time PCR assay of TNF-α and IL-6 mRNA amount in the cells transfected as inaand then stimulated with 100 ng ml−1LPS or 10 μg ml−1CpG for 3 h. Data are shown as mean±s.d. (n=3). **P<0.01 (Student’st-test). Similar results were obtained in three independent experiments. (d,e) Immunoblot of phosphorylated and total ERK1/2, p38, JNK and NF-κB p65 in cells transfected as inaand then stimulated with 10 μg ml−1CpG (d) or 100 ng ml−1LPS (e) for indicated time. Similar results were obtained in three independent experiments. (f) Luciferase assay of activation of Elk1 in HEK293T cells transfected with 50 ng MyD88-expressing plasmid, 100 ng Elk1 luciferase reporter plasmid, 2.5 ng pTK-Renilla-luciferase, together with 0, 25 or 50 ng of MEKK2- or mutant MEKK2ΔC-expressing plasmid. Luciferase activity was measured and normalized by Renilla luciferase activity. Data are shown as mean±s.d. (n=4) of one typical experiment (**P<0.01, Student’st-test). Similar results were obtained in three independent experiments. Figure 4: MEKK2 mediates ERK1/2 activation in TLR signalling. ( a ) Immunoblot assay of MEKK2 expression in mouse peritoneal macrophages transfected with 30 nM control siRNA (Ctrl) or MEKK2 siRNA. Similar results were obtained in three independent experiments. ( b ) ELISA assay of TNF-α and IL-6 in the supernatants of the cells transfected as in a and then stimulated with 100 ng ml −1 LPS or 10 μg ml −1 CpG for 6 h. Data are shown as mean±s.d. ( n =3). ** P <0.01 (Student’s t -test). Similar results were obtained in three independent experiments. ( c ) Real-time PCR assay of TNF-α and IL-6 mRNA amount in the cells transfected as in a and then stimulated with 100 ng ml −1 LPS or 10 μg ml −1 CpG for 3 h. Data are shown as mean±s.d. ( n =3). ** P <0.01 (Student’s t -test). Similar results were obtained in three independent experiments. ( d , e ) Immunoblot of phosphorylated and total ERK1/2, p38, JNK and NF-κB p65 in cells transfected as in a and then stimulated with 10 μg ml −1 CpG ( d ) or 100 ng ml −1 LPS ( e ) for indicated time. Similar results were obtained in three independent experiments. ( f ) Luciferase assay of activation of Elk1 in HEK293T cells transfected with 50 ng MyD88-expressing plasmid, 100 ng Elk1 luciferase reporter plasmid, 2.5 ng pTK-Renilla-luciferase, together with 0, 25 or 50 ng of MEKK2- or mutant MEKK2ΔC-expressing plasmid. Luciferase activity was measured and normalized by Renilla luciferase activity. Data are shown as mean±s.d. ( n =4) of one typical experiment (** P <0.01, Student’s t -test). Similar results were obtained in three independent experiments. Full size image Stk38 inhibits MEKK2 expression To investigate the role of Stk38 in MEKK2-dependent ERK1/2 activation, we observed the effect of Stk38 overexpression on MEKK2-induced Elk1 luciferase reporter gene expression. As anticipated, overexpression of Stk38 inhibited MEKK2-mediated Elk1 luciferase reporter gene expression ( Fig. 5a ). Overexpression of MEKK2 leads to activation of MEKK2 itself. Although activated MEKK2 ran with lower migration, inactive MEKK2 ran with higher migration in SDS–polyacrylamide gel electrophoresis (SDS–PAGE). Interestingly, we found that the expressions of both active and inactive MEKK2 were reduced by Stk38 overexpression ( Fig. 5b ). Consistently, compared with that in wild-type control cells, MEKK2 expression in Stk38-deficient macrophages was increased ( Fig. 5c ), demonstrating that Stk38 negatively regulated MEKK2-mediated signalling by inhibiting MEKK2 expression. As a protein kinase, Stk38 was reported to phosphorylate p21 and decrease expression of p21. K118A mutation disrupted Stk38 kinase activity and led to p21 accumulation [23] . To investigate whether Stk38 inhibited MEKK2 expression via its kinase activity as in the case of p21, we constructed Stk38K118A mutant-expressing plasmid ( Fig. 5d ). As shown in Fig. 5e , kinase-inactive Stk38K118A inhibited MEKK2 expression as efficiently as wild-type Stk38, indicating that Stk38 inhibited MEKK2 expression through a kinase activity-independent mechanism. In addition to central kinase catalytic domain, Stk38 has a short N-terminal and a hydrophobic motif-containing C-terminal ( Fig. 5d ). Deletion of C-terminal partially impaired the capability of Stk38 to decrease MEKK2 expression. However, deletion of both the N- and C-terminal made Stk38 completely lose the capability to decrease MEKK2 expression, suggesting that both of the N-terminal and C-terminal of Stk38 were required for Stk38 to inhibit MEKK2 expression ( Fig. 5e ). 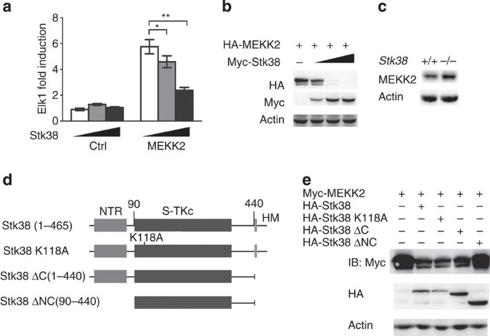Figure 5: Stk38 inhibits MEKK2 expression. (a) Luciferase assay of activation of Elk1 in HEK293T cells transfected with 50 ng MEKK2-expressing plasmid, 100 ng Elk1 luciferase reporter plasmid, 2.5 ng pTK-Renilla-luciferase and 0, 100 or 200 ng of Stk38-expressing plasmid. Luciferase activity was measured and normalized by Renilla luciferase activity. Data are shown as mean±s.d. (n=4) of one typical experiment (**P<0.01, Student’st-test). Similar results were obtained in three independent experiments. (b) Immunoblot assay of MEKK2 expression in HEK293T cells transfected with MEKK2-expressing plasmid and increased amount of Stk38-expressing plasmid. Similar results were obtained in three independent experiments. (c) Immunoblot assay of MEKK2 expression in wild-type (WT) and Stk38-deficient macrophages. Similar results were obtained in three independent experiments. (d) Schematic diagram of wild-type and mutant Stk38. Numbers in parentheses indicate amino acids included in the constructs. (e) Immunoblot (IB) assay of MEKK2 expression in HEK293 cells transfected with MEKK2-expressing plasmid together with wild-type or mutant Stk38-expressing plasmids. Similar results were obtained in three independent experiments. Figure 5: Stk38 inhibits MEKK2 expression. ( a ) Luciferase assay of activation of Elk1 in HEK293T cells transfected with 50 ng MEKK2-expressing plasmid, 100 ng Elk1 luciferase reporter plasmid, 2.5 ng pTK-Renilla-luciferase and 0, 100 or 200 ng of Stk38-expressing plasmid. Luciferase activity was measured and normalized by Renilla luciferase activity. Data are shown as mean±s.d. ( n =4) of one typical experiment (** P <0.01, Student’s t -test). Similar results were obtained in three independent experiments. ( b ) Immunoblot assay of MEKK2 expression in HEK293T cells transfected with MEKK2-expressing plasmid and increased amount of Stk38-expressing plasmid. Similar results were obtained in three independent experiments. ( c ) Immunoblot assay of MEKK2 expression in wild-type (WT) and Stk38-deficient macrophages. Similar results were obtained in three independent experiments. ( d ) Schematic diagram of wild-type and mutant Stk38. Numbers in parentheses indicate amino acids included in the constructs. ( e ) Immunoblot (IB) assay of MEKK2 expression in HEK293 cells transfected with MEKK2-expressing plasmid together with wild-type or mutant Stk38-expressing plasmids. Similar results were obtained in three independent experiments. Full size image Stk38 promotes Smurf1-mediated polyubiquitination of MEKK2 E3 ubiquitin ligase Smurf1 inhibits MEKK2 expression by catalysing K48-linked ubiquitination of MEKK2 (ref. 24 ). We explored whether Stk38 affected the regulation of MEKK2 expression by Smurf1. In HEK293T cells, Stk38 or Smurf1 overexpression alone inhibited MEKK2 expression ( Fig. 6a ). Interestingly, combination of Stk38 and Smurf1 overexpression much more efficiently inhibited MEKK2 expression than Stk38 or Smurf1 alone, demonstrating that Stk38 and Smurf1 synergistically inhibited MEKK2 expression. Carboxyl terminus of Hsc70-interacting protein (CHIP) is also an ubiquitin E3 ligase that promotes the K48-linked ubiquitination and degradation of MEKK2 (ref. 25 ). However, combination of Stk38 and CHIP overexpression failed to inhibit MEKK2 expression more efficiently ( Supplementary Fig. 8 ). To reveal the underlying mechanism by which Stk38 inhibited MEKK2 expression synergistically with Smurf1, we tested whether Stk38 promoted Smurf1-mediated MEKK2 ubiquitination. MEKK2, Smurf1 and haemagglutinin (HA)-tagged ubiquitin-expressing plasmids were transfected into HEK293T cells in the absence or presence of Stk38. After 24 h, MEKK2 was immune-precipitated, and ubiquitination of MEKK2 was detected with anti-HA antibody and K48-ubiquitin-specific antibody. As shown in Fig. 6b , Stk38 increased total ubiquitination and K48-linked ubiquitination of MEKK2 in the presence of Smurf1. C699A mutation of Smurf1 made Smurf1 lose its ubiquitin ligase activity [26] . Stk38 overexpression did not affect MEKK2 ubiquitination in the presence of Smurf1C699A ( Fig. 6c ), demonstrating that Stk38 increased MEKK2 ubiquitination in Smurf1-dependent manner. The ability of Stk38 to regulate MEKK2 ubiquitination was further investigated by in vitro ubiquitin ligase activity assay. As shown in Fig. 6d , Smurf1 recombinant protein catalysed ubiquitination of MEKK2 in vitro . Addition of Stk38 recombinant protein increased MEKK2 ubiquitination, confirming that Stk38 could promote Smurf1-mediated MEKK2 ubiquitination. 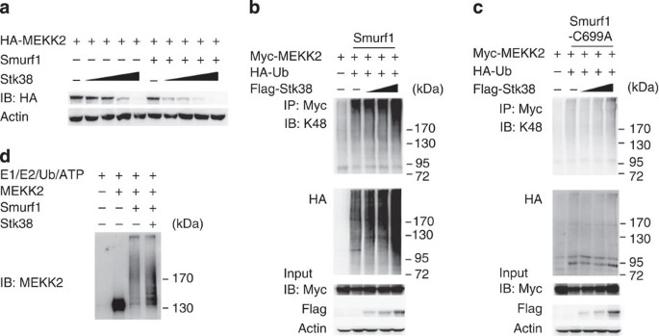Figure 6: Stk38 promotes Smurf1-mediated MEKK2 polyubiquitination. (a) Immunoblot (IB) of MEKK2 expression in HEK293T cells transfected with various combinations (above lanes) of plasmids encoding HA-MEKK2, Smurf1 and Stk38. Similar results were obtained in three independent experiments. (b,c) IB of K48 and total ubiquitination of MEKK2 in HEK293T cells transfected with various combinations (above lanes) of plasmids encoding Myc-MEKK2, HA-ubiquitin (HA-Ub), Stk38-Flag, wild-type Smurf1 (b) or mutant Smurf1(C699A) (c), treated with proteasome inhibitors MG132 and MG115, followed by denaturation-immunoprecipitation (IP) with anti-Myc and IB analysis with anti-HA or antibody specific for K48-linked ubiquitin (K48). Input MEKK2, Stk38 and Actin in whole-cell lysates were blotted with anti-Myc, anti-Flag and anti-actin antibodies (bottom three blots). Similar results were obtained in three independent experiments. (d) IB analysis of MEKK2 incubatedin vitrowith Smurf1 and Stk38 recombinant proteins and the full complement of ubiquitination reaction components. Similar results were obtained in three independent experiments. Figure 6: Stk38 promotes Smurf1-mediated MEKK2 polyubiquitination. ( a ) Immunoblot (IB) of MEKK2 expression in HEK293T cells transfected with various combinations (above lanes) of plasmids encoding HA-MEKK2, Smurf1 and Stk38. Similar results were obtained in three independent experiments. ( b , c ) IB of K48 and total ubiquitination of MEKK2 in HEK293T cells transfected with various combinations (above lanes) of plasmids encoding Myc-MEKK2, HA-ubiquitin (HA-Ub), Stk38-Flag, wild-type Smurf1 ( b ) or mutant Smurf1(C699A) ( c ), treated with proteasome inhibitors MG132 and MG115, followed by denaturation-immunoprecipitation (IP) with anti-Myc and IB analysis with anti-HA or antibody specific for K48-linked ubiquitin (K48). Input MEKK2, Stk38 and Actin in whole-cell lysates were blotted with anti-Myc, anti-Flag and anti-actin antibodies (bottom three blots). Similar results were obtained in three independent experiments. ( d ) IB analysis of MEKK2 incubated in vitro with Smurf1 and Stk38 recombinant proteins and the full complement of ubiquitination reaction components. Similar results were obtained in three independent experiments. Full size image Then the association between Stk38 and Smurf1 in TLR9 signalling was investigated by immunoprecipitation experiments. As shown in Fig. 7a , Stk38 constitutively associated with Smurf1 in macrophages, and the association could be enhanced by CpG stimulation. When incubated in vitro , Stk38 recombinant protein was efficiently co-precipitated with Smurf1 by Smurf1-specific antibody ( Fig. 7b ), demonstrating that Stk38 directly interacted with Smurf1. To evaluate more fully the binding between Stk38 and Smurf1, we constructed a series of mutant Smurf1-expressing plasmids to map the domains required for Smurf1 to interact with Stk38 ( Fig. 7c ). Smurf1ΔC2 expressed truncated Smurf1 lacking N-terminal 138 amino-acid residues, which contained C2 domain. Smurf1ΔHECT lacked C-terminal HECT domain. Smurf1ΔWW lacked the intermediate WW domain. Although Stk38 could be immune-precipitated with wild-type Smurf1, it could not be immune-precipitated with any of the three truncated mutants ( Fig. 7d ). This result suggested that each of the three domains was required for the interaction between Smurf1 and Stk38. Similarly as many other E3 ubiquitin ligases, activation of Smurf1 was dependent on ubiquitination of itself [27] . Thus, we detected the effect of Stk38 on Smurf1 ubiquitination. As shown in Fig. 7e , overexpression of Stk38 increased total ubiquitination as well as K63- and K48-linked Smurf1 ubiquitination. Mutant Stk38K118A also increased Smurf1 ubiquitination, suggesting Stk38 promoted Smurf1 ubiquitination independently of its kinase activity. To validate whether Smurf1 inhibited TLR9 responses, we observed the effect of Smurf1 RNA interfering on CpG-induced proinflammatory cytokine production. Smurf1-specific siRNA could efficiently inhibit endogenous Smurf1 expression in mouse peritoneal macrophages ( Fig. 7f ). Smurf1 knockdown increased CpG-induced TNF-α and IL-6 production in mouse peritoneal macrophages ( Fig. 7g ), demonstrating that Smurf1 was a negative regulator of TLR9 responses. These results demonstrated that Stk38 inhibited TLR9 signalling by promoting Smurf1-mediated MEKK2 ubiquitination. 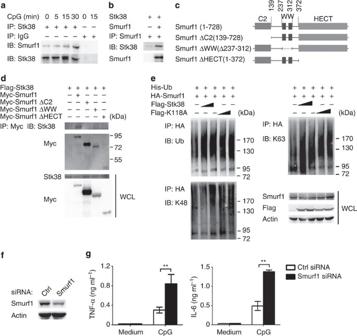Figure 7: Stk38 promotes Smurf1 ubiquitination. (a) Immunoblot (IB) analysis of proteins immune-precipitated (IP) with Stk38-specific antibody or immunoglobulin G (IgG) from lysates of mouse peritoneal macrophages stimulated with 10 μg ml−1CpG for indicated times. Similar results were obtained in three independent experiments. (b) Immunnoblot of Stk38 protein incubated with Smurf1 and then IP with Smurf1-specific antibodies. Similar results were obtained in three independent experiments. (c) Schematic diagram of wild-type and mutant Smurf1. Numbers in parentheses indicate amino acids included in construct. (d) HEK293T cells were transfected with Stk38-expressing plasmid together with Myc-tagged wild-type and mutant Smurf1-expressing plasmids followed by immune-precipitation with anti-Myc antibody. Stk38 and Smurf1 were blotted with Stk38-specific and anti-Myc antibodies. Similar results were obtained in three independent experiments. (e) IB of K48-linked, K63-linked and total ubiquitination of Smurf1 in HEK293T cells transfected with various combinations (above lanes) of plasmids encoding His-ubiquitin (His-Ub), HA-Smurf1, Flag-Stk38 and Flag-Stk38K118A, treated with MG132 and MG115, followed by denaturation-IP with anti-HA. Input Smurf1, Stk38, Stk38K118A and actin in whole-cell lysates (WCL) were blotted with anti-Smurf1, Flag or Actin antibody. Similar results were obtained in three independent experiments. (f) IB assay of Smurf1 in mouse peritoneal macrophages transfected with 30 nM control small RNA (Ctrl) or Smurf1-specific siRNA. Similar results were obtained in three independent experiments. (g) ELISA assay of TNF-α and IL-6 in the supernatants of the cells transfected as infand then stimulated with 10 μg ml−1CpG for 6 h. Data are shown as mean±s.d. (n=3). **P<0.01 (Student’st-test). Similar results were obtained in three independent experiments. Figure 7: Stk38 promotes Smurf1 ubiquitination. ( a ) Immunoblot (IB) analysis of proteins immune-precipitated (IP) with Stk38-specific antibody or immunoglobulin G (IgG) from lysates of mouse peritoneal macrophages stimulated with 10 μg ml −1 CpG for indicated times. Similar results were obtained in three independent experiments. ( b ) Immunnoblot of Stk38 protein incubated with Smurf1 and then IP with Smurf1-specific antibodies. Similar results were obtained in three independent experiments. ( c ) Schematic diagram of wild-type and mutant Smurf1. Numbers in parentheses indicate amino acids included in construct. ( d ) HEK293T cells were transfected with Stk38-expressing plasmid together with Myc-tagged wild-type and mutant Smurf1-expressing plasmids followed by immune-precipitation with anti-Myc antibody. Stk38 and Smurf1 were blotted with Stk38-specific and anti-Myc antibodies. Similar results were obtained in three independent experiments. ( e ) IB of K48-linked, K63-linked and total ubiquitination of Smurf1 in HEK293T cells transfected with various combinations (above lanes) of plasmids encoding His-ubiquitin (His-Ub), HA-Smurf1, Flag-Stk38 and Flag-Stk38K118A, treated with MG132 and MG115, followed by denaturation-IP with anti-HA. Input Smurf1, Stk38, Stk38K118A and actin in whole-cell lysates (WCL) were blotted with anti-Smurf1, Flag or Actin antibody. Similar results were obtained in three independent experiments. ( f ) IB assay of Smurf1 in mouse peritoneal macrophages transfected with 30 nM control small RNA (Ctrl) or Smurf1-specific siRNA. Similar results were obtained in three independent experiments. ( g ) ELISA assay of TNF-α and IL-6 in the supernatants of the cells transfected as in f and then stimulated with 10 μg ml −1 CpG for 6 h. Data are shown as mean±s.d. ( n =3). ** P <0.01 (Student’s t -test). Similar results were obtained in three independent experiments. Full size image Signal transductions of TLR family members activate different immune responses. Illuminating the mechanisms by which TLR4 and TLR9 signal transductions are differently regulated is helpful in understanding how TLR4 and TLR9 trigger different immune responses. Compared with TLR4 signal transduction, which has been intensively investigated, less is known about the mechanisms by which TLR9 activates downstream MAPK and NF-κB pathways. In the present study, we showed that MEKK2 and Stk38 preferentially regulated signal transduction of TLR9 rather than TLR4 in macrophages. MEKK2 was reported to be phosphorylated following LPS stimulation, and overexpression of MEKK2(S519A) mutant could inhibit LPS-induced Elk1 luciferase reporter gene expression, indicating that MEKK2 might play a role in TLR4 signalling. However, overexpression of MEKK2 did not affect LPS-induced cathelicidin-related antimicrobial peptide gene expression in mast cells [9] . In our experiments, MEKK2 knockdown only slightly inhibited LPS-induced ERK1/2 activation, suggesting that endogenous MEKK2 might be dispensable or redundant for ERK1/2 activation in TLR4 signalling. In contrast, MEKK2 knockdown significantly inhibited CpG-induced ERK1/2 activation and suppressed CpG-induced TNF-α and IL-6 production, identifying MEKK2 as a novel important mediator in TLR9 signal transduction. It remains unclear why MEKK2 was differently required for LPS- and CpG-induced ERK1/2 activation. It has been proven that Tpl2 is indispensable for LPS-induced ERK1/2 activation [4] . However, Tpl2 deficiency completely blocked LPS-induced ERK1/2 activation but did not affect CpG-induced ERK1/2 activation in mouse peritoneal macrophages [28] . These results indicate that TLR4 and TLR9 use different signal transduction mediators to activate downstream MAPKs. Stk38-deficient mice produced much more proinflammatory cytokine following E. coli infection. Stk38-deficient mice showed increased lethality than control wild-type mice following E. coli infection and CLP surgery, suggesting that Stk38 played an important role in protecting host from bacterial infection, possibly by limiting excessive inflammatory cytokine production and inflammatory injuries. Both of Stk38 knockdown and Stk38 knockout increased CpG-induced proinflammatory cytokine production without affecting LPS- and LTA-induced inflammatory cytokine production, demonstrating that Stk38 protected host by negatively regulating TLR9-mediated innate immunity. In this study, E. coli infection and CLP surgery models were used to investigate the role of Stk38 in sepsis. Human sepsis patients usually are treated with continual fluid administration, antibiotics and other supportive care. It is worthy to study whether Stk38 deficiency affects the sepsis when the mice are provided with supportive therapy. E3 ubiquitin ligase Smurf1 regulated MEKK2 ubiquitination and negatively regulated MEKK2 expression. The ubiquitin ligase activity of Smurf1 could be regulated by its interaction with other proteins such as Cdh1 and CKIP-1 (refs 27 , 29 ). Our results demonstrated that Stk38 directly interacted with Smurf1 and promoted Smurf1-mediated MEKK2 ubiquitination. The interaction between Stk38 and Smurf1 also increased ubiquitination of Smurf1 itself, suggesting that the interaction between Smurf1 and Stk38 positively regulated the ligase activity of Smurf1. In a recent study, Smurf1 was reported to promote TGF-β-induced MyD88 ubiquitination and inhibit LPS-induced NF-κB activation in the presence of exogenous TGF-β [30] . Differently, we found that Smurf1 RNA interfering could increase CpG-induced proinflammatory cytokine production in macrophages even in the absence of exogenous TGF-β. Given that MEKK2, the substrate of Smurf1, was required for TLR9-induced ERK1/2 activation, it was reasonable to deduce that Smurf1 could modulate TLR9 signalling by regulating MEKK2 expression. Taken together, our study demonstrated that MEKK2 was required for TLR9-mediated ERK1/2 activation and proinflammatory cytokine production in macrophages. Stk38 negatively regulated TLR9 responses in macrophages by directly interacting with Smurf1, promoting Smurf1-mediated K48-linked ubiquitination of MEKK2 and inhibiting MEKK2 expression. Stk38-deficient mice were more susceptible to bacterial infection-induced sepsis. These results demonstrated that Stk38 was an important negative regulator of TLR9-mediated innate immunity in macrophages and was necessary for protecting host from TLR9-mediated inflammation. Mice Mice heterozygous for Stk38 (TF2907) on 129/SvEv-C57BL/6 genetic background were purchased from Taconic Biosciences (Hudson). The mice were bred in specific pathogen-free conditions and intercrossed to get homozygous knockout mice and wild-type control littermates. Cells from female littermates (6–8 weeks old) were subjected to in vitro experiments. C57BL/6 mice (6–8 weeks old) were obtained from Joint Ventures Sipper BK Experimental Animal Company. All studies were conducted in accordance with the National Institute of Health Guide for the Care and Use of Laboratory Animals with approval of the Scientific Investigation Board of Second Military Medical University, Shanghai. Cell culture and reagents The RAW264.7 and HEK293T cell lines were purchased from American Type Culture Collection. All cells were maintained in DMEM (Hyclone) with 10% (vol/vol) FBS. LPS (437628) was from Calbiochem. LTA (L2515) was from Sigma. Phosphorothioate-modified CpG ODN (5′- TCCATGACGTTCCTGATGCT -3′) was synthesized by Sangon Biotech Co. (Shanghai, China). Antibodies specific for Myc tag (sc-40), Actin (sc-1616), MEKK2 (sc-1088), Smurf1 (sc-100616), Stk38 (sc-46183), p38 (sc-535), ERK1/2 (sc-93), JNK (sc-7345), p65 (sc-109) were from Santa Cruz Biotechnology. Antibodies specific for phosphorylated ERK1/2 (9101), phosphorylated p38 (9216), phosphorylated p65 (3033), phosphorylated JNK (9251), K48-Ubiquitin (4289), K63-Ubiquitin (5621) and Flag tag (8146) were from Cell Signaling Technology. These antibodies were applied at the dilution 1:1,000. Anti-HA tag (H3663) antibody was from Sigma and applied at the dilution 1:5,000. Recombinant MEKK2 (M0324) was from Sigma, Smurf1 (ab95928) from Abcam and Stk38 (TP304133) from Origene. Ubiquitin, E1 and E2 proteins were from Boston Biochem. Peritoneal macrophages preparation Thioglycollate-elicited mouse peritoneal macrophages were isolated as previously described [31] .C57BL/6 mice (6–8 weeks old) were intraperitoneally injected with 2 ml3% sodiumthioglycollate (Sigma) solution each. Three days later, cells in the abdominal cavity were collected by lavaging with 10–15 ml DMEM without FBS and centrifugated. Cells were seeded and maintained in DMEM with 10% (vol/vol) FBS. After removing the floating cells 24 h later, adhered peritoneal macrophages were subjected for further experiments. Plasmid constructs The pGFP-V-RS vectors expressing shRNA targeting mouse Stk38 (5′- GCCATACCTTCGTACATGAAAGCAGCAAA -3′) and control shRNA were from OriGene. Elk1 luciferase reporter Vector (LR0019) was from Panomics. MyD88-expressing vector was described previously [32] . Human cDNA encoding MEKK2 was amplified from mRNA of Hela cells by reverse transcription–PCR. pCMV6-XL5-Stk38 vector expressing human Stk38 and pCMV6-Kan/Neo-Smurf1 vector expressing mouse Smurf1 were purchased from Origene, and used as templates to amplify cDNA expressing full-length and truncated Stk38 or Smurf1 that were cloned into pCMV-Myc or pCMV-HA expression vector (Clontech) to construct Myc- or HA-tagged MEKK2, Stk38- and Smurf1-expressing plasmids. HA-CHIP-expressing plasmid was a gift from Mingjin Yang (Institute of Immunology, Second Military Medical University) [33] . Flag-Stk38 construct was a gift from Xiaojian Wang (Institute of Immunology, Zhejiang University). RNA interfering For transient knockdown, small RNA was transfected into thioglycollate-elicited mouse peritoneal macrophages with INTERFERin according to the manufacturer’s instructions (Polyplus). For stable knockdown, plasmids expressing shRNA were transfected into RAW264.7 macrophages. The cells were selected with puromycin (5 μg ml −1 ) and pooled for further experiments. MEKK2-specific interfering RNAssiRNA (5′- GGUCCAUUAUUUGCAUAGUTT -3′) and siRNA2 (5’- UAUUUCUCUUGAUUCUUGGTT -3′) were used to inhibit MEKK2 expression. Smurf1-specific interfering RNA (5′- GGAGGAAGGUUUGGACUAUTT -3′) was used to inhibit Smurf1 expression. ‘non-sense’ sequence (5′- UUCUCCGAACGUGUCACGUTT -3′) (Genepharma) was used as control siRNA. Control Non-target siRNA, Stk38 and Stk38L On-target siRNA were from Dharmacon. Quantitative reverse transcription–PCR Total RNA was extracted with RNA extraction kit and cDNA was synthesized using reverse transcriptase M-MLV (Takara) according to the manufacturer’s instructions. Real-time PCR was performed with a SYBR RT-PCR kit (Takara) on LightCycler (Roche). The primers used were β-Actin-F (5′- AGTGTGACGTTGACATCCGT -3′), β-Actin-B (5′- GCAGCTCAGTAACAGTCCGC -3′), TNF-α-F (5′- AAGCCTGTAGCCCACGTCGTA -3′), TNF-α-B (5′- GGCACCACTAGTTGGTTGTCTTTG -3′), IL-6-F (5′- TAGTCCTTCCTACCCCAATTTCC -3′) and IL-6-B (5′- TTGGTCCTTAGCCACTCCTTC -3′). Detection of cytokine production The concentrations of TNF-α and IL-6 in culture supernatants or serum were measured with ELISA kits according to the manufacturer’s instructions (eBioscience). Assay of luciferase reporter gene expression HEK293T cells were co-transfected with Elk1 activity luciferase reporter plasmid, pRL-TK-Renilla-luciferase plasmid and indicated amount of MyD88-, Stk38- or MEKK2-expressing plasmids. After 24 h, luciferase activity in the cell lysates were measured with a Dual-Luciferase Reporter Assay system according to the manufacturer’s instructions (Promega). The luciferase activity was normalized for transfection efficiency by division with Renilla luciferase activity. Immunoprecipitation and immunoblot analysis The experiments were carried out as previously described [31] . Briefly, cells were lysed with M-PER Protein Extraction Reagent (Pierce) supplemented with protease inhibitor cocktail, and protein concentrations of the extracts were measured with BCA assay according to the manufacturer’s instructions (Pierce). Equal amounts of extracts were used for immunoprecipitation with antibodies and Protein G magnetic beads (Millipore), or loaded for SDS–PAGE, transferred onto nitrocellulose membranes and then blotted with indicated antibodies. Finally, signal intensity was determined using the Tanon 5200S Chemiluminescent Imaging System (Tanon). Images have been cropped for presentation. Full-size images are presented in Supplementary Fig. 9 . Detection of protein ubiquitination HEK293T cells were transfected with plasmids expressing MEKK2, Stk38, Smurf1 and ubiquitin. After 12 h, cells were treated with proteasome inhibitors MG132 and MG115 for another 12 h. Samples were collected and boiled for 10 min after adding 1% SDS. The cell lysate was diluted to 0.1% SDS with lysis buffer. Protein concentrations of the extracts were measured, and equal amounts of extracts were used for immunoprecipitation of target protein. Prepared samples were resolved on 6% SDS–PAGE and transferred to nitrocellulose membrane. Detection of polyubiquitination was performed with indicated antibodies [34] . For in vitro ligase activity assay, recombinant MEKK2, Smurf1, Stk38 and ubiquitination-associated proteins were mixed in reaction buffer with ATP as indicated. All tubes were incubated at 30 °C for 2 h. Reaction was terminated by adding sample-loading buffer and boiled for 10 min. Samples were resolved on 6% SDS–PAGE [35] . Establishment of E. coli infection model Mice of 6–8 weeks old were challenged with live E. coli intraperitoneally (5 × 10 7 E. Coli , strain O111:B4, per mouse). Survivals of mice were monitored for 2 days. Establishment of CLP-induced sepsis CLP of mice was performed as previously described [36] . Mice were completely anaesthetized with sevoflurane for inhalation (Hengrui) mixed with oxygen via anaesthetic evaporator VP300 (Yi’an) before and during the surgery. After anaesthetized, the central abdominal laparotomy was performed with an incision of 1–1.5 cm. The cecum was exteriorized and about 50% was ligated. Then one hole was made in the cecum with a 22-G needle at the end. The mice were resuscitated with 1 ml pre-warmed sterile physiologic saline solution by subcutaneous injection after surgery. All mice were given free access to food and water after recovery from anaesthesia. Mice were monitored for clinic score and survival for 5 days. Clinical symptoms were scored on a scale of 0–5 (ref. 37 ). Statistical analysis The statistical significance of comparisons between two groups was determined with Student’s t -test. Survival curves were estimated using the method of Kaplan and Meier and statistical analysis of the curves was performed by Gehan–Breslow–Wilcoxon test. P values of less than 0.05 were considered statistically significant. How to cite this article: Wen, M. et al . Stk38 protein kinase preferentially inhibits TLR9-activated inflammatory responses by promoting MEKK2 ubiquitination in macrophages. Nat. Commun. 6:7167 doi: 10.1038/ncomms8167 (2015).